Tracking lithium transport and electrochemical reactions in nanoparticles Expectations for the next generation of lithium batteries include greater energy and power densities along with a substantial increase in both calendar and cycle life. Developing new materials to meet these goals requires a better understanding of how electrodes function by tracking physical and chemical changes of active components in a working electrode. Here we develop a new, simple in-situ electrochemical cell for the transmission electron microscope and use it to track lithium transport and conversion in FeF 2 nanoparticles by nanoscale imaging, diffraction and spectroscopy. In this system, lithium conversion is initiated at the surface, sweeping rapidly across the FeF 2 particles, followed by a gradual phase transformation in the bulk, resulting in 1–3 nm iron crystallites mixed with amorphous LiF. The real-time imaging reveals a surprisingly fast conversion process in individual particles (complete in a few minutes), with a morphological evolution resembling spinodal decomposition. This work provides new insights into the inter- and intra-particle lithium transport and kinetics of lithium conversion reactions, and may help to pave the way to develop high-energy conversion electrodes for lithium-ion batteries. Lithium-ion batteries are the preferred energy storage devices for portable electronics and will have an important role in large-scale applications, such as electric vehicles and grid-scale storage [1] . The transition from portable electronics, which typically last 2–3 years, to vehicles and grid, with expected lifetime greater than 10 years, will require substantial improvements in calendar and cycling life. In addition, automotive applications require at least a two-fold improvement in energy and power densities. One of the promising classes of electrode materials that could meet these requirements is lithium conversion compounds, which have the advantage of accommodating more than one lithium per transition metal, boasting high theoretical capacities [2] , [3] , [4] , and in some cases, exhibit excellent capacity retention. A recent study of lithium conversion in the FeF 2 cathode offered the first experimental evidence of the formation of a conductive iron network, [5] which may provide the pathway for electron transport necessary for reversible lithium cycling [2] , [4] , [6] , [7] . However, these electrodes are typically plagued by poor cycling rate and a large cycling hysteresis [8] , [9] . Improvements will require a better understanding of the phase nucleation and evolution, electron and ion transport, and reaction kinetics, which are difficult to determine by ex-situ measurements. Most of the available in-situ techniques, such as those based on hard X-ray scattering, are suited for studying bulk electrodes and have inadequate spatial resolution for exploring nanoscale morphological and structural changes, and determining where and how new phases nucleate and propagate [10] , [11] . Transmission electron microscopy (TEM), capable of exceptional spatial resolution has, until recently, been unsuitable for these studies due to issues associated with the limited space between the objective lens pole pieces, low electron transparency and an incompatibility of the liquid electrolyte with the high vacuum environment. A few recent attempts to circumvent these issues involved sealed liquid cells or open cells with an ionic liquid (low vapour pressure) or solid electrolyte [12] , [13] , [14] , [15] , [16] . However, these approaches are often unsuitable for high-resolution studies of nanoparticles because of reduced electron transparency (as a result of the thick window) and/or the requirement for special electrode morphologies (for example, nanowires/rods, or thin films). Importantly, these techniques are mostly incapable of tracking the structural and chemical evolution occurring in the electrodes during charge/discharge. Here we develop a new, simple in-situ electrochemical cell for the TEM by adapting a commercially available biasing system, as illustrated in Fig. 1a . A lithium metal counter electrode was applied to a sharp tungsten tip that was attached to a piezo-driven biasing-probe built into the TEM–scanning tunnelling microscopy sample stage (Nanofactory Instruments AB). The lithium electrochemical reaction with FeF 2 , which occurs via a conversion process (FeF 2 +2Li + +2e − →2LiF+Fe), was investigated using FeF 2 -C nanocomposite electrodes, with FeF 2 nanoparticles supported on carbon. The evolution of the electrode undergoing the conversion reaction was captured over a range of length scales—capturing changes in the composite (micron-scale) and within an individual particle (sub-nanometre scale), via real-time TEM imaging, electron diffraction (ED) and electron energy-loss spectroscopy (EELS) recorded at sub-second temporal resolution. First-principles calculations and phase-field simulations were employed to elucidate the origin of the observed morphological and phase evolution, and the underlying mechanisms involved in the electrochemical conversion reaction. In this study, direct experimental observation, supported by computation, reveals that the lithium conversion is initiated at the surface and then propagates into the bulk with a morphological evolution resembling spinodal decomposition, resulting in the formation of a network of interconnected Fe nanoparticles (1–3 nm) within the amorphous LiF. 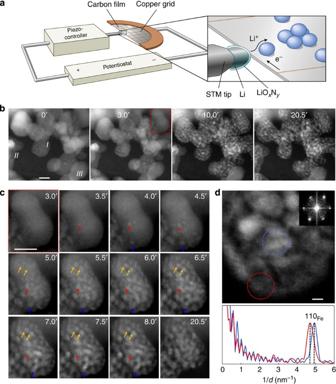Figure 1: Lithium conversion of FeF2monitored in real time. See alsoSupplementary Figs S1 and 2, andSupplementary Movies 1and2. (a) Schematic of the electrochemical cell used forin-situTEM measurements. (b) Time-lapse images from a collection of particles that react with lithium coming from the lower right. The reaction proceeds immediately in region (I), but is delayed and absent in regions (II) and (III), respectively. Scale bar, 10 nm. (c) Morphological evolution of a single FeF2nanoparticle, revealing the rapid formation of ultrafine (sub-nm) Fe particles on the surface, followed by gradual formation of larger ones (1–3 nm) within the domain of the original FeF2particle (arrows used to identify specific Fe particles). Scale bar, 10 nm. (d) Lattice image of Fe particles converted from a single FeF2particle (top), aligned along the zone [−1,1,1] according to the fast Fourier transform (FFT) pattern (inset), and intensity profiles of the FFT patterns (bottom) from the Fe lattice in the near-surface region (red circle) and central region (blue circle). Scale bar, 2 nm. Figure 1: Lithium conversion of FeF 2 monitored in real time. See also Supplementary Figs S1 and 2 , and Supplementary Movies 1 and 2 . ( a ) Schematic of the electrochemical cell used for in-situ TEM measurements. ( b ) Time-lapse images from a collection of particles that react with lithium coming from the lower right. The reaction proceeds immediately in region ( I ), but is delayed and absent in regions ( II ) and ( III ), respectively. Scale bar, 10 nm. ( c ) Morphological evolution of a single FeF 2 nanoparticle, revealing the rapid formation of ultrafine (sub-nm) Fe particles on the surface, followed by gradual formation of larger ones (1–3 nm) within the domain of the original FeF 2 particle (arrows used to identify specific Fe particles). Scale bar, 10 nm. ( d ) Lattice image of Fe particles converted from a single FeF 2 particle (top), aligned along the zone [−1,1,1] according to the fast Fourier transform (FFT) pattern (inset), and intensity profiles of the FFT patterns (bottom) from the Fe lattice in the near-surface region (red circle) and central region (blue circle). Scale bar, 2 nm. Full size image Lithium reaction with individual nanoparticles The FeF 2 -C composite electrodes were made with as-synthesized 10–20 nm FeF 2 particles dispersed on thin carbon films and further incorporated into the setup illustrated in Fig. 1a for the in-situ TEM measurements. The real-time morphological changes occurring during lithiation were recorded in Supplementary Movies 1 and 2 , and annular dark-field (ADF) images ( Fig. 1b ). The reaction front propagates extremely fast and sweeps across the collection of particles in region I within a few seconds ( Supplementary Movie 1 ). In contrast, the reaction is delayed (by about 10 min) in region II , and does not occur at all in region III , even after more than 20 min. The reduced activity in these regions is likely due to poor contact between particles and the current collector, which inhibits ion and electron transport. On the other hand, this observation confirms that the observed morphological changes are due to the conversion reaction rather than beam-induced phase decomposition that may also occur under intense electron irradiation [17] . The electrochemical conversion of a single particle is shown in the time-lapse images in Fig. 1c , revealing a rapid surface reaction leading to the formation of small, sub-nanometre Fe particles, followed by the reaction in the bulk, resulting in slightly larger (1–3 nm) Fe particles. The lithiation under an external bias clearly indicates two different timescales for inter- and intra-particle Li + transport (see also Supplementary Movie 2 and Supplementary Fig. S1 ). The Li ions appear to move quickly via surface diffusion along the carbon film and FeF 2 particles, and then penetrate into the bulk at a much slower rate. There is no observable coarsening of the newly formed Fe nanoparticles throughout the conversion period ( Fig. 1b and Supplementary Movie 1 ). This observation suggests an immediate decomposition reaction that occurs locally, and that the LiF may be effective at blocking interparticle Fe diffusion and thereby preventing coarsening. It is also interesting to note that the lattice of the Fe particles in the near-surface region is slightly larger (by ~4%) compared with the lattice of the slightly larger particles in the centre as seen in the fast Fourier transform of Fig. 1d . This type of lattice expansion may be attributed to a nano-size effect, as similar expansions have been observed in metal nanoparticles with particle dimensions in a similar range [18] , [19] . The Fe crystallites, converted within the same FeF 2 particle, tend to be interconnected and aligned in the same crystallographic orientation ( Fig. 1d ), which has also been observed in previous ex-situ TEM experiments [5] . The distinct morphological feature of Fe in the near-surface region, that is, forming a chain-like structure ( Supplementary Fig. S3 ), suggests that the phase-decomposition process may occur spontaneously on the surface and propagate into the core. The reaction within individual particles is surprisingly fast, complete within 3–12 min (listed in Supplementary Table S1 ), and is equivalent to a discharge rate of 5–20 C in a full battery. Slow kinetics is believed to be intrinsic and insurmountable in conversion electrodes, which would limit their use in real batteries [6] . However, these real-time observations challenge this traditional belief and indicate that rapid cycling rates may be achieved by engineering an electrode with active nanoparticles directly connected to the current collector [9] , rather than the traditional method of preparing heterogeneous nanocomposite electrodes, which often leads to agglomerates of active materials [3] , [5] , [20] . A large volume expansion (41–57%) is observed in the particles during the reaction as the low-density LiF phase is formed, filling in the space around the Fe particles. As the expected volume expansion is only 21%, based on the crystalline densities these results suggest that the newly formed Fe and LiF nanoparticles are not densely packed. Given the low sputtering cross-section of iron at 200 kV (~4.1 barn calculated using the Mott model), little damage is expected to the iron [21] . However, a fraction of the LiF could be destroyed via quick radiolysis. Quasi in-situ measurements were performed with the beam off during the reaction, and with the beam on briefly to record images and spectra of particles immediately before and after lithiation. The TEM images ( Supplementary Fig. S4a,b ) show that the size and morphology of the Fe particles formed during the quasi in-situ measurements are nearly identical to those formed during the in-situ measurements. The EELS spectra and elemental maps ( Supplementary Fig. S4c,d ) acquired from the lithiated particles clearly show the presence of LiF and a high spatial correlation with the iron nanoparticles. Lithium transport in thin films In-situ measurements were also made on FeF 2 -C film electrodes, composed of a single layer of contiguous FeF 2 nanoparticles (10–20 nm in diameter) on a 10-nm-thick carbon film ( Fig. 2a ), which provides the media for tracking the Li transport and a quantitative measure of the propagation of the reaction front. In the ADF images, the bright contrast of the Fe nanoparticles formed on the surface, best seen in the boundary region ( Fig. 2b ), was used to identify the reaction front, which was observed to propagate rapidly across the film (from lower right to upper left). A plot of the position of the reaction front (distance from the lower right corner, d ) versus time, t ( Fig. 2c ), was fit to a power law, t n with n <1. Rapid Li + surface diffusion clearly has an important role in the advancement of the front. Nevertheless, individual grains undergo a slow reaction process as shown by the time-lapse images in Supplementary Fig. S5 . These observations are consistent with those in Fig. 1 . 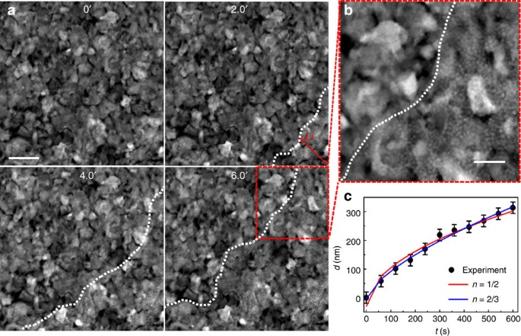Figure 2: Lithium conversion in FeF2film showing the rapid propagation of the reaction front. See alsoSupplementary Movie 3. (a) Representative time-lapse images showing the movement of the reaction front across the area, as indicated by the white dashed lines. Scale bar, 50 nm. (b) A magnified view showing the boundary defined with the bright contrast of the newly formed Fe nanoparticles. Scale bar, 20 nm. (c) Distance,d, of the reaction front propagation, measured from the lower right corner, as a function of time,t, (solid circles), fit with a power law, ~tn, forn=1/2 (red), 2/3 (blue). The error bars come from the uncertainties in defining the boundaries (~20 nm). Figure 2: Lithium conversion in FeF 2 film showing the rapid propagation of the reaction front. See also Supplementary Movie 3 . ( a ) Representative time-lapse images showing the movement of the reaction front across the area, as indicated by the white dashed lines. Scale bar, 50 nm. ( b ) A magnified view showing the boundary defined with the bright contrast of the newly formed Fe nanoparticles. Scale bar, 20 nm. ( c ) Distance, d , of the reaction front propagation, measured from the lower right corner, as a function of time, t , (solid circles), fit with a power law, ~ t n , for n =1/2 (red), 2/3 (blue). The error bars come from the uncertainties in defining the boundaries (~20 nm). Full size image Structural evolution by in-situ ED A series of ED patterns were recorded, at a frequency of two patterns per second, to monitor the structural evolution of FeF 2 particles during the electrochemical reaction. Upon lithiation, the intensity of the diffraction rings associated with the FeF 2 phase decreases along with a corresponding increase in those associated with the Fe phase, as illustrated in Fig. 3 . The Bragg rings associated with the Fe phase are broad and diffuse because of the small crystallite size ( Supplementary Fig. S6 ). In the intensity profile ( Fig. 3b ), there is no noticeable shift in the position of the FeF 2 peaks, even at the early stage of the reaction, providing direct evidence of little-to-no lithium insertion during the reaction process. The position and intensity of the Fe (110) peak were estimated through fitting, by which the Fe (110) peak was separated from the neighbouring FeF 2 (210) peak ( Supplementary Fig. S6c ). It should be noted that the contribution from the Fe (110) peak becomes dominant with lithiation, due to ~60 times greater Bragg intensity than the FeF 2 (210) peak, as predicted by electron structure factor calculations ( Supplementary Table S2 ). The Fe (110) peak initially appears at lower angles (with respect to that of the bulk) and increases in intensity and shifts to higher angles during the electrochemical reaction ( Fig. 3c ). This shift is consistent with a reaction where small (sub-nanometre) Fe particles, with a slightly larger lattice, nucleate first in the near-surface region ( Fig. 1d ), followed by the formation of larger (1–3 nm) particles with a ‘bulk-like’ lattice parameter. This type of lattice expansion was also recently observed in Fe nanoparticles converted from Fe 2 O 3 ( [22] ). 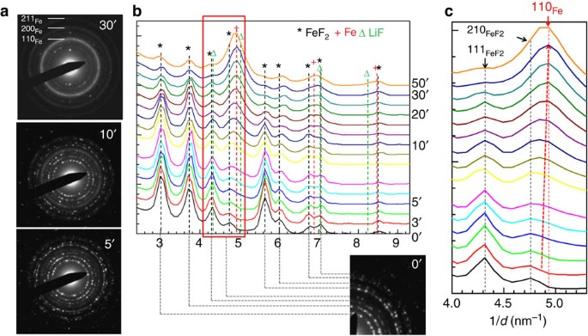Figure 3: Structural evolution of FeF2nanoparticles byin-situED. See alsoSupplementary Movie 4. (a) Representative ED patterns recorded at 5, 10 and 30 min. (b) Integrated intensity from a selection of ED patterns recorded at different time (labelled on the right side). The correspondence of the peaks with the specific rings in the ED pattern is illustrated for the first pattern (at 0 min). (c) A magnified view showing the growth of Fe phase at the expense of the FeF2phase and the shift of the Fe (110) peak upon lithiation, which is illustrated by a red dashed line (see alsoSupplementary Fig. S6cfor changes in peak position and intensity determined from peak fitting). The expected positions of peaks associated with the three different phases were indicated with different markers: *FeF2, +Fe and ΔLiF. Figure 3: Structural evolution of FeF 2 nanoparticles by in-situ ED. See also Supplementary Movie 4 . ( a ) Representative ED patterns recorded at 5, 10 and 30 min. ( b ) Integrated intensity from a selection of ED patterns recorded at different time (labelled on the right side). The correspondence of the peaks with the specific rings in the ED pattern is illustrated for the first pattern (at 0 min). ( c ) A magnified view showing the growth of Fe phase at the expense of the FeF 2 phase and the shift of the Fe (110) peak upon lithiation, which is illustrated by a red dashed line (see also Supplementary Fig. S6c for changes in peak position and intensity determined from peak fitting). The expected positions of peaks associated with the three different phases were indicated with different markers: *FeF 2 , +Fe and ΔLiF. Full size image Chemical evolution by in-situ EELS The spectra in the low-loss region, containing the Li K- and Fe M 23 -edges were acquired continuously to monitor the chemical evolution upon lithium conversion ( Supplementary Movie 5 ). The representative time-lapse spectra shown in Fig. 4a show a gradual fading of the shoulder in the Fe M 23 peak (at about 55 eV) and growth of the Li K-edge (at about 62 eV) as a result of conversion from FeF 2 to Fe and LiF. Supplementary TEM images and ED patterns were also recorded from the FeF 2 particles in the pristine and fully lithiated states ( Fig. 4b ), providing further information on the phase transition and morphological change. The gradual formation of LiF during the conversion was clearly detected by in-situ EELS measurements, but the diffraction peaks associated with this phase were hardly detectable (inset of Fig. 4b ), similar to the observation in Fig. 3 . If LiF is present as a crystalline phase, the strongest scattering ring, LiF (200), would have an amplitude similar to that of the Fe (200) peak ( Supplementary Table S2 ). The absence of the LiF Bragg rings suggests that this phase may be amorphous when it initially forms, which is consistent with the prediction by molecular dynamics simulations [23] . The disordered LiF phase may be more ionically conductive than crystalline LiF, [23] but it is not thermodynamically stable at room temperature and crystallizes over time. This may also explain the presence of crystalline LiF in the fully lithiated FeF 2 electrodes examined ex-situ . 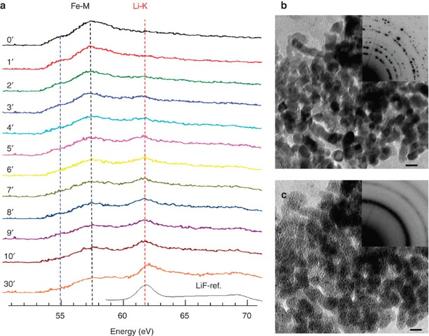Figure 4: Chemical evolution of FeF2nanoparticles byin-situEELS. See alsoSupplementary Movie 5. (a) Time-lapse EELS spectra showing the evolution of the chemical states of Fe and Li, as indicated by the variations in the fine structure of the Fe M23- and Li K-edges during the conversion process. Reference Li K-edge spectrum (LiF-ref.) recorded from LiF compound is shown at the bottom to confirm the formation of LiF, by the characteristic peaks at about 62 and 69 eV. (b,c) Bright-field TEM images and ED patterns (inset) of the FeF2nanoparticles in the pristine and fully lithiated states, respectively. Scale bar, 20 nm. [5] Figure 4: Chemical evolution of FeF 2 nanoparticles by in-situ EELS. See also Supplementary Movie 5 . ( a ) Time-lapse EELS spectra showing the evolution of the chemical states of Fe and Li, as indicated by the variations in the fine structure of the Fe M 23 - and Li K-edges during the conversion process. Reference Li K-edge spectrum (LiF-ref.) recorded from LiF compound is shown at the bottom to confirm the formation of LiF, by the characteristic peaks at about 62 and 69 eV. ( b , c ) Bright-field TEM images and ED patterns (inset) of the FeF 2 nanoparticles in the pristine and fully lithiated states, respectively. Scale bar, 20 nm. Full size image In-situ TEM offers a unique glimpse of the nanoscale phase transformations that occur during electrochemical conversion reactions. The processes observed here pose a true challenge to theoretical interpretation, as they take place at length scales too large for direct atomistic simulations, but also too small for a rigorous continuum treatment. Although the converting system is a nanoscale mixture of insulating and metallic phases containing many interfaces, phase stability based on a homogeneous free-energy description should nevertheless provide some guidance. 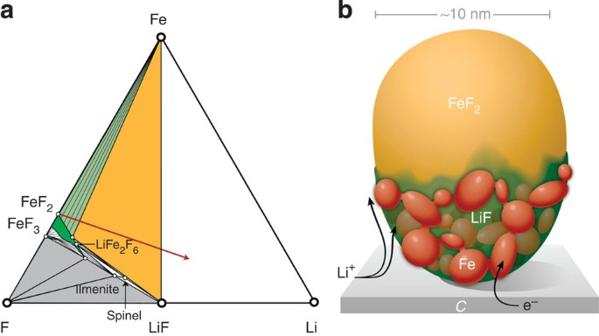Figure 5: Possible reaction paths in FeF2. (a) Fe-F-Li phase diagram informed by extensive first-principles calculations of known and candidate structures. (b) Schematic illustration of the propagation of reaction front through a single FeF2particle via a ‘layer-by-layer’ process and possible pathway for electron and Li+transport. Figure 5a shows a phase diagram in the ternary Fe-F-Li composition space informed by a large number of first-principles calculations of known and likely structures for this system based on density functional theory (DFT) [24] . The various experimental observations during the conversion reaction are inconsistent with the minimum free-energy path (that is, equilibrium phase sequence dictated by the phase diagram), which predicts that sub-stoichiometric tri-rutile LiFe 2 F 6 should form first through a displacement reaction followed by a conversion to Fe and LiF (as indicated by the arrow). The predicted voltage curve for this equilibrium path ( Supplementary Fig. S8 ) is substantially higher than that measured experimentally [5] . It should be noted that the predicted voltage is a lower bound for the equilibrium path, as we used an energy for pure Fe that accounted for the contribution of surface energies at the nanoscale [24] . In addition, the Fe 3+ (expected for LiFe 2 F 6 ) was not identified by in-situ EELS measurements ( Fig. 4 ), and the predicted variation of the lattice parameter of rutile Li x Fe 1-x F 2 , of about 12% ( Supplementary Fig. S9 ), was not detected in the diffraction measurements ( Fig. 3 ). This suggests that the reaction follows one of several possible metastable (non-equilibrium) paths. Figure 5: Possible reaction paths in FeF 2 . ( a ) Fe-F-Li phase diagram informed by extensive first-principles calculations of known and candidate structures. ( b ) Schematic illustration of the propagation of reaction front through a single FeF 2 particle via a ‘layer-by-layer’ process and possible pathway for electron and Li + transport. Full size image One possibility is the direct Li intercalation into FeF 2 until the structure becomes highly supersaturated with Li upon which it decomposes into LiF and Fe. The voltage predicted under this scenario ( Supplementary Fig. S8 ) is significantly lower than that of the equilibrium path and is also more consistent with the measurements [5] . However, although Li is predicted to have a very high mobility within rutile FeF 2 , direct intercalation into FeF 2 would lead to energetically undesirable Fe +1 along with a continuous variation in the lattice parameter, which was not observed experimentally. In fact, DFT calculations predict that the rutile crystal structure becomes unstable above a low Li insertion threshold, relaxing to highly deformed structures that have little in common with the original rutile structure. This suggests that Li insertion into rutile FeF 2 may be accompanied by the amorphization of the host, thereby making it invisible to diffraction probes and explaining the absence of lattice parameter variations with increasing Li content. The supersaturated amorphous phase can then decompose at a slower rate, requiring the redistribution of more sluggish Fe and F, not unlike a spinodal decomposition reaction. The resemblance of the meso-structure observed in TEM to spinodal decomposition is striking, as illustrated by the projection of a continuum simulation of spinodal decomposition within an ellipsoidal particle, Supplementary Fig. S10 , simulated based on the Cahn–Hilliard equation [25] with a smoothed boundary method [26] . Nevertheless, this mechanism, which involves the amorphization of the nanoparticles, fails to provide an explanation for the coherent nature of the interconnected Fe network, unless this coherency forms at a later stage, either due to physical rotation of the Fe nanoparticles as they impinge (to eliminate the cost of grain boundary energy) or through a recrystallization mechanism. An alternative mechanism could be driven by interface processes. Although fluorine mobility within the rutile-like structure is lower than that of Li or Fe ( Supplementary Fig. S11 ), the reaction could still be controlled by fluorine redistribution with most of the F transport occurring along the interfaces that emerge as the two-phase mixture (LiF+Fe) grows at the expense of FeF 2 . Such a mechanism would also be consistent with an interconnected network of nanometre-sized Fe particles, as it would essentially be a nanoscale manifestation of a eutectoid reaction. Furthermore, the extraction of F from rutile FeF 2 at its surface could result in the collapse of the body-centred tetragonal Fe sublattice of the rutile structure to form the body-centred cubic crystal structure of pure Fe. This would result in a unique crystallographic orientation of the resultant Fe relative to the original FeF 2 host and could explain the coherency of the Fe network. Although many questions remain around the true mechanisms behind this conversion reaction, our understanding is distinctly different from what has been speculated about conversion reactions in the absence of these unique in-situ TEM studies. Our observations reveal that Li ions move quickly along the surface, and then penetrate into the bulk of FeF 2 particles at a much slower rate. The reaction path is complex, involving interplay of ion and electron transport dynamics within a nanoscale mixture of multiple phases. A combination of real-time observations with DFT calculations and phase-field simulations seems to suggest a ‘layer-by-layer’ propagation process in the conversion reaction, as illustrated in Fig. 5b . Diffusion of Li into the bulk is prohibited, but may be allowed locally in the near-surface region, leading to the supersaturation of a thin layer and immediate spinodal-like phase decomposition. The newly formed Fe nanoparticles and three-phase (Fe/LiF/FeF 2 ) interfaces provide a pathway for electron and lithium transport into the particle. In contrast to the fast lithiation reaction in intercalation materials that may allow bulk Li diffusion, the conversion reaction is considerably slower, taking a few minutes for an ~10-nm particle, and has strong dependence on the particle size, which may be attributed to the ‘layer-by-layer’ propagation process. These results, from a model conversion system (FeF 2 ), may shed new light on nanocomposite formation in other metal fluorides and other types of conversion materials (for example, oxides, nitrides and sulphides) [27] . The size and distribution of the nanophases directly impacts the electrochemical performance of these electrodes. The beautiful aspect of the electrochemical conversion process is that it leads to exceptionally fine phase formation, including metals with crystallites <3 nm, through a self-limited intrinsic reaction. It is worth noting that the electrochemical conversion reaction may also be a useful procedure for preparing unique nanostructured networks, suitable for a variety of applications including catalysis and photoconversion [28] . Although this present study is a distinct step towards understanding the process of electrochemical conversion, additional studies are necessary to better understand how the transport properties of electrons and atomic species influence cycling hysteresis, and the formation and evolution of nanocrystallites. Importantly, the newly developed in-situ cell and methodologies provide an opportunity to track the phase evolution and the formation of intermediate phases (if they occur) during the discharge and charge reactions [5] , [24] . Future studies will focus on the reconversion (charge) reaction in an attempt to gain new insights into the cycling hysteresis that plague most conversion electrodes. In-situ TEM experiments An in-situ cell (shown in Fig. 1a ) suitable for TEM was developed and used for studying the electrochemical reaction of FeF 2 nanoparticles. The samples were directly loaded onto 10 nm thick amorphous carbon films supported on the copper half-grids. The carbon film has a similar role as the carbon black used in general FeF 2 -C electrodes, acting as a support, and also the media for electron and ion transport. A thin layer of lithium metal (as the counter electrode) was coated onto a sharp tungsten tip that was attached to a piezo-driven biasing-probe built into the TEM–scanning tunnelling microscopy sample stage (Nanofactory Instruments AB). All of the components were assembled in an Argon glove box and then transferred into the TEM column using an Ar-filled bag. As illustrated in Fig. 1a , a full battery was built in the TEM by connecting the Li-coated tungsten tip with the carbon support using the piezo controller. The battery was composed of a copper grid (current collector), FeF 2 -C (cathode) and Li metal (anode). A thin passivation layer of LiN x O y on the surface of the Li acted as the solid electrolyte [29] , [30] . The biasing probe was connected to the carbon and the reaction was only initiated by applying a negative bias typically at a value of 2 V or higher; correspondingly, a low current across the whole electrode was measured, mostly below 60 nA. No reaction or current flow occurred before applying the bias or with a lower biasing potential. In-situ TEM images, ED patterns and EELS spectra were recorded at 200 kV in a JEOL2100F microscope equipped with a Gatan image filter spectrometer. The energy resolution was ~1.1 eV, as judged by the full-width at half-maximum of the zero-loss peak. Spectra were recorded either in a scanning TEM (STEM) mode for local analysis, or parallel-beam TEM mode from many particles. ADF–STEM imaging (with z -contrast) was employed in this experiment to provide good contrast for the small Fe particles. High-resolution ADF–STEM images were also acquired from the lithiated samples in a dedicated STEM machine (Hitachi 2,700D, with a probe aberration-correction system), to identify the crystallographic orientations of the converted Fe nanoparticles. During the in-situ TEM measurements, electron beam irradiation was minimized by opening the valve only during the data acquisition. The alignment was performed in a sacrificial region and the measurements were taken on a nearby region that had not been previously exposed to the beam (this procedure was followed in all the in-situ measurements). The total dose was minimized by using the lowest possible magnification and beam current, with some sacrifice in resolution and contrast. Diffraction patterns and EELS spectra were recorded in TEM mode with a spread beam. To examine the irradiation effect on the electrochemical reaction of FeF 2 particles, ‘ quasi in-situ ’ measurements were also made, with the electron beam off during the reaction, and compared with the in-situ measurements. Fabrication of FeF 2 nanoparticles and thin films The FeF 2 nanoparticles were obtained by a solution process from iron metal and fluorosilicic acid solutions (H 2 SiF 6 ), as described in [31] . The as-prepared FeF 2 nanoparticles were 10–20 nm in diameter, mostly with well-defined nearly spherical or ellipsoidal shapes. The FeF 2 films were fabricated by thermal evaporation in high vacuum, with a base pressure of 10 −7 Torr, at both room temperature and elevated temperature (measured on the substrate). The films were deposited on amorphous 10-nm-thick carbon films. The size of the FeF 2 grains varied and was strongly dependent on the temperature of the substrate, from 2 to 3 nm at 25 °C, to 10–20 nm at 300 °C ( Fig. 2 ). Electron structure factor calculations The electron structure factor was calculated by where f j , r j and B j are the electron atomic scattering amplitude, the atomic position and the Debye-Waller factor, respectively, g is the reciprocal vector, and s is the scattering vector, s =g/2. In a kinematical approximation (a good approximation for the powder ED of nanoparticles), the intensity of the reflection is where γ is the relativistic constant ( γ =1.3914 for an accelerating voltage of 200 kV), and Ω is the volume of the unit cell. For powder electron diffraction, the integrated ring intensity is where M g is the multiplicity of the reflection g . Supplementary Table S2 lists the values for F g and R g . First-principles electronic structure calculations Our first-principles calculations extended those of Doe et al . [24] to establish phase equilibria in the Li-Fe-F ternary composition space. The calculations were also performed to estimate relative mobilities between Li, Fe and F in the various stable compounds. These first-principles calculations were performed using DFT, with generalized gradient approximation parameterized by Perdew and Wang [32] , as implemented with the Vienna ab initio Simulation Package [33] . Core states were treated with the projector-augmented wave method [34] , [35] using the valence state 3 p 1 3 d 7 4 s 1 for Fe, 1 s 1 2 s 1 2 p 1 for Li and 2 s 2 2 p 5 for F. An energy cutoff value of 550 eV was used. Brillioun zone integration was performed on k -point meshes that are equivalent or denser than a 6 × 6 × 6 k -point mesh for rutile-unit cell and perovskite unit cell and on an 11 × 11 × 11 mesh for structures based on an face-centered cubic fluorine lattice to obtain a k -point convergence of less than 5 meV per atom. All cell parameters and atom positions were allowed to relax fully to achieve energy minimization for each structure. Ferromagnetic, spin-polarized calculations were implemented in all structures containing Fe, as both FeF 2 and FeF 3 are known to exhibit antiferromagnetic properties below the Neel temperature ( T N ), 79 K and 363 K, respectively [36] , [37] . To determine phase stability in the Li-Fe-F ternary, we calculated the energies of ~1,360 different compounds. Of this total, ~890 of them were rutile-based structures (including trirutile-based structures), ~65 perovskite-based, ~5 cryolite-based, ~25 spinel-based, ~25 ilmenite-based, ~320 face-centered cubic fluorine sublattice-based and ~30 hexagonal close-packed fluorine sublattice-based. In the construction of the Li-Fe-F equilibrium phase diagram, the Fe reference state was raised by 1 eV to account for several effects [24] . The first is that in generalized gradient approximation calculations, there is an energy discrepancy between the localized d -states of the ionic iron in the fluoride and the delocalized states in metallic iron [24] . Another effect to consider is that although the calculations may represent bulk materials, the conversion reactions are only feasible in nano-sized particles. Therefore, an adjustment must also be made to account for the difference between bulk and nano materials (estimated for a 3.7 nm particle) [24] . The nudged-elastic band method as implemented in Vienna ab initio Simulation Package was used to calculate the migration barriers of Li and Fe. Supercells containing 12 rutile FeF 2 unit cells (2 a × 2 a × 3 c ), where a and c are the primitive unit-cell lattice parameters, were used with a 3 × 3 × 2 k -point grid. All nudged-elastic band calculations were performed at constant volume, after having fully relaxed the initial state of the cell, and a decreased energy cutoff value of 400 eV. A total of five images were interpolated between the initial and final states of the migration barrier. The migration barrier of F was calculated by taking the energy difference between the initial and a final state (thereby giving a lower bound for its migration barrier) within a supercell of four trirutile LiFe 2 F 6 unit cells (2 a × 2 a × 1 c ) on a 4 × 4 × 4 k -point grid. The Li migration barrier in FeF 2 along the empty tunnels in the (001) direction ( Supplementary Fig. S7 ) is about 90 meV, which would indicate high lithium mobility. A slightly more realistic scenario where the valence of Fe is preserved to be 2+ is a structure with a dilute concentration of Fe replaced by Li (Li 2 Fe 23 F 48 ). In this case, the Li migration barrier in the empty tunnels is 170 meV, suggesting high lithium mobility in partially converted structures. Within a structure of the same composition, the Fe migration barrier amounts to 450 meV. The F migration barrier in an even further converted structure, namely trirutile (Li 8 Fe 16 F 47 ), turns out to be much higher, around 900 meV ( Supplementary Fig. S11 ). Phase-field simulation The phase-field method is based on the dynamics driven by the reduction of the total free energy, which leads to the evolution of the order parameter. The order parameter can be either conserved (for example, concentration) or non-conserved (for example, crystallographic orientation). For a simple, conserved system, which can be described by the Cahn–Hilliard equation, the total free energy is approximated by [25] where f ( C ) is the bulk free-energy function in terms of the order parameter C , and κ is the gradient energy coefficient. We employed the smoothed boundary method [26] to simulate the phase separation confined in the interior of an ellipsoidal particle. The region where phase separation occurs is defined by a domain parameter that specifies the domain in which the evolution equation is solved; ψ =1 inside the domain and ψ =0 outside the domain. The evolution equation is then reformulated to To confine the region in which phase separation takes place to an ellipsoidal shell to simulate the conversion of FeF 2 , the domain parameter profile was calculated by where is the scaled distance to the centre of the ellipsoid particle, located at the origin, R o is the parameter that determines the size of the ellipsoidal particle, R i is the parameter that determines the size of the inner surface below which the concentration remains constant at the initial value, and ς is used to control the thickness of the region between ψ =1 and ψ =0. Equation (5) is dimensionless and was discretized using the second-order central differencing scheme in space within a domain containing 90 × 90 × 128 Cartesian grid points and a first-order Euler explicit scheme in time. The grid spacing and time step of Δ x =1 and Δ t =5 × 10 −3 , respectively, were used. The domain parameter was defined by equation 6 with l a = l b =2, l c =3, and R o =18. Four values of R i were examined (18, 13, 9 and 0) such that the 4 sets of simulations represent varying thickness of regions undergoing spinodal decomposition. We set ς to be 0.5 for the domain parameter profile, and the gradient energy coefficient κ to be 1.0 to ensure that there were sufficient number of grid points in the interfacial region for numerical accuracy. The initial order parameter for the simulation was set as C ( x , t =0)=0.5+0.005η( x ), where η( x ) is given by a random number between −1 and 1 at each grid point, which gives a noise with an amplitude of 1% of the average concentration. How to cite this article: Wang, F. et al . Tracking lithium transport and electrochemical reactions in nanoparticles. Nat. Commun. 3:1201 doi: 10.1038/ncomms2185 (2012).